Determining volcanic eruption styles on Earth and Mars from crystallinity measurements Both Earth and Mars possess different styles of explosive basaltic volcanism. Distinguishing phreatomagmatic eruptions, driven by magma–water interaction, from ‘magmatic’ explosive eruptions (that is, strombolian and plinian eruptions) is important for determining the presence of near-surface water or ice at the time of volcanism. Here we show that eruption styles can be broadly identified by relative variations in groundmass or bulk crystallinity determined by X-ray diffraction. Terrestrial analogue results indicate that rapidly quenched phreatomagmatic ejecta display lower groundmass crystallinity (<35%) than slower cooling ejecta from strombolian or plinian eruptions (>40%). Numerical modelling suggests Martian plinian eruptive plumes moderate cooling, allowing 20–30% syn-eruptive crystallization, and thus reduce the distinction between eruption styles on Mars. Analysis of Mars Curiosity rover CheMin X-ray diffraction results from Gale crater indicate that the crystallinity of Martian sediment (52–54%) is similar to pyroclastic rocks from Gusev crater, Mars, and consistent with widespread distribution of basaltic strombolian or plinian volcanic ejecta. Predominant styles of volcanic eruptions on Mars are likely to differ as compared with those on Earth, with theoretical considerations suggesting that highly explosive, finer grained and more widely distributed mafic volcanism may be more prevalent in the Martian environment [1] , [2] , [3] , [4] , [5] . Despite the absence of a present-day liquid hydrosphere on Mars, magma–water driven (that is, phreatomagmatic) eruptions are also possible through interaction with ice or subsurface water [6] . Both direct and indirect observations of volcanic deposits on Mars are now possible, but unequivocally constraining Martian eruption styles remains challenging. Factors affecting explosive mafic volcanism on Earth, such as overburden pressure in the magma chamber, geometry of the conduit, viscosity of the magma (influenced by microlite crystallization and bubble content), and volatile content and degassing history [7] , [8] , [9] are analogous to those operating on Mars, despite differences in eruption scale between these two rocky planets. Widespread and layered equatorial deposits including the Medusae Fossae Formation and kilometre-thick Vallis Marineris interior deposits have been postulated to at least partially comprise volcanic ash or pyroclastic flow deposits from explosive mafic eruptions [10] , [11] , [12] . The Mars Science Laboratory (MSL) Curiosity rover will have a unique opportunity to test models of layered deposit formation during its future traverse of Mount (Mt.) Sharp (officially termed Aeolis Mons), a 5.3-km-tall sequence of layered deposits in the centre of Gale Crater, that fits the criteria for these types of deposits [13] and potentially contains a continuous marker bed that is traceable around much of Mt. Sharp [14] . To date, Curiosity has encountered mainly volcaniclastic and isochemically altered basaltic sediments along its traverse to Yellowknife Bay [15] . Given the high likelihood that Curiosity will continue to encounter volcanically derived deposits, we present here a novel methodology to distinguish between types of mafic explosive eruptions on rocky planets (for example, plinian, strombolian and phreatomagmatic). We have explored the hypothesis that groundmass crystallinity ( C gm ) measured by X-ray diffraction (XRD) analysis may be correlated to eruption style and potentially used as a remote tool for constraining Martian eruption dynamics. C gm is defined as the volume percent of a crystalline component in a mixed crystalline–amorphous material, which is a function of magma cooling history. Traditionally, the microlite content in basaltic volcanic rocks has been linked to pre-eruptive factors such as magma ascent rate and degassing history, particularly in the shallow conduit [16] , [17] . However, crystallization of basaltic melt can occur extremely rapidly, and significant groundmass crystallization may continue after eruption within more slowly cooling clasts [18] . Magma–water interaction driven by marine, ground- or surficial water results in extremely rapid cooling (>10 6 K s −1 ; ref. 19 ), whereas studies of magmatic airfall products indicate maximum cooling rates of ≤10 K s −1 (refs 18 , 20 ). Phreatomagmatism favours the formation of quenched basaltic glass, withgroundmass crystallinities significantly lower than those observed in air-cooled magmas. Here we show how groundmass crystallinities, and by extension random bulk (that is, whole rock) crystallinities, determined from XRD analysis of a suite of terrestrial basaltic deposits enable development of a criterion for constraining eruption styles. We demonstrate from analysis of terrestrial volcanism that products of phreatomagmatic eruptions predominantly have groundmass and bulk (groundmass+phenocryst) crystallinities below ~40%, whereas crystallinities from strombolian and plinian basaltic eruptions are typically >40%. Remote determination of crystallinity of volcanic samples by the CheMin instrument, an XRD instrument on board the MSL Curiosity rover [21] , therefore provides a novel approach for identifying magma–water interactions in the record of explosive volcanism on Mars, and potentially evaluating the evolution of the Martian hydrosphere as preserved in the volcanic record. 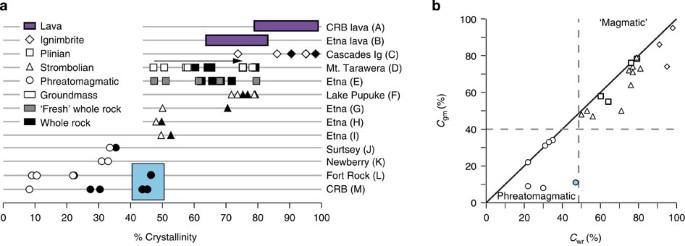Figure 1: Crystallinity of natural samples. (a) Calculated crystallinity of volcanic deposits from XRD analysis plotted versus sample location. Samples are broadly organized by volcanic eruption style. The range of groundmass crystallinity (Cgm) of lava flows are indicated by purple bars. Increasing crystallinity with clast size for the 1886 Mt. Tarawera plinian eruption is indicated by a black arrow. The blue box indicates phreatomagmatic whole-rock samples that are severely altered/weathered. (b) Comparison of hand-pickedCgmto bulk ‘random sample’ crystallinity (Cwr). Dashed grey lines delineate the approximate division between phreatomagmatic and ‘magmatic’ eruption styles. The severely altered/weathered whole-rock Fort Rock (Sample L) phreatomagmatic material containing fresh groundmass glass is indicated in blue. Sample locations and descriptions are keyed toTable 1by their ID labels indicated in parentheses. Eruption style from crystallinity measurements Eruptive styles of the explosive basaltic samples we have analysed include deposits from phreatomagmatic, basaltic plinian and strombolian (including fire fountaining) eruptions ( Figs 1 and 2 ; and Table 1 ). Basaltic lava flows from the Columbia River flood basalts and Mt. Etna were also analysed to help verify the analytical technique ( Fig. 1 and Table 1 ). Crystallinity is determined for both groundmass ( C gm ) and random bulk sampling ( C wr ) when possible. XRD crystallinity measurements qualitatively agree with textural observations, both macroscopically and from back-scatter electron imaging, which shows that the analysed material ranges from translucent and glassy (8% crystallinity; Columbia River basalt hyaloclastite) to dull (>50% crystallinity; Tarawera) ( Figs 1 and 2 and Table 1 ). Prior investigations of this technique have documented the correlation between XRD results and crystallinity obtained from back-scatter electron image processing [22] . Figure 1: Crystallinity of natural samples. ( a ) Calculated crystallinity of volcanic deposits from XRD analysis plotted versus sample location. Samples are broadly organized by volcanic eruption style. The range of groundmass crystallinity ( C gm ) of lava flows are indicated by purple bars. Increasing crystallinity with clast size for the 1886 Mt. Tarawera plinian eruption is indicated by a black arrow. The blue box indicates phreatomagmatic whole-rock samples that are severely altered/weathered. ( b ) Comparison of hand-picked C gm to bulk ‘random sample’ crystallinity ( C wr ). Dashed grey lines delineate the approximate division between phreatomagmatic and ‘magmatic’ eruption styles. The severely altered/weathered whole-rock Fort Rock (Sample L) phreatomagmatic material containing fresh groundmass glass is indicated in blue. Sample locations and descriptions are keyed to Table 1 by their ID labels indicated in parentheses. 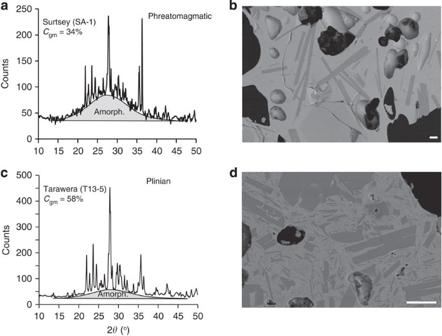Figure 2: Phreatomagmatic versus plinian eruptive products. Representative groundmass diffraction patterns (a,c) and scanning electron microscope back-scatter images (b,d) for a phreatomagmatic eruption (Surtsey) and basaltic plinian eruption (Tarawera). Grey regions ina,crepresent the area under the diffraction pattern associated with the amorphous (Amorph., glass) component from 10–40° 2θ. Bragg peaks, identified here by X-ray count rates above background, represent the diffraction of X-rays off various lattice planes within minerals in the sample, and therefore represent the crystalline component. White scale bars, 20 μm (b,d). Full size image Figure 2: Phreatomagmatic versus plinian eruptive products. Representative groundmass diffraction patterns ( a , c ) and scanning electron microscope back-scatter images ( b , d ) for a phreatomagmatic eruption (Surtsey) and basaltic plinian eruption (Tarawera). Grey regions in a , c represent the area under the diffraction pattern associated with the amorphous (Amorph., glass) component from 10–40° 2 θ . Bragg peaks, identified here by X-ray count rates above background, represent the diffraction of X-rays off various lattice planes within minerals in the sample, and therefore represent the crystalline component. White scale bars, 20 μm ( b , d ). Full size image Table 1 Sample descriptions and crystallinity measurements. Full size table The crystallinity of phreatomagmatic materials (negligible to moderate weathering) investigated is generally low, ranging from 8 to 35% ( Fig. 1 ). This contrasts with other ‘magmatic’ eruption styles that have C wr and C gm values >40% (47–80%). Lava crystallinity is generally high, with C wr from 77 to 98% ( C gm >64%; Fig.1 ). Groundmass crystallinities are a function of cooling rate; thin, smaller lava flows cool more rapidly and, as such, have lower C gm than slowly cooled massive lava flows. Particle size can variably affect interpretation of the crystallinity results. For example, groundmass chips were hand-picked from 125 and 250 μm sieve fractions to avoid microphenocrysts in one tuffaceous deposit (Fort Rock, OR). From the 125- to 250-μm-size fractions, we observed an increase in C gm from 9 to 22%. This difference may reflect more complete exclusion of microphenocrysts in the 125-μm-sieved fraction, and may imply that the smaller, hand-picked size fraction more accurately represents C gm . A bulk crystallinity ( C wr ) measurement of the same 125-μm-sieved fraction as the groundmass separate (that is, comparable to the Curiosity rover sampling methodology [21] ) has the same crystallinity ( C wr =22%) as the whole rock—note that this is also the same value as C gm from the 250-μm-sieved fraction. The identical C wr between the 125-μm-size fraction and the bulk rock analysis may imply that, unlike C gm , C wr is relatively insensitive to the analysed size fraction. Clast size controls much of the variation seen in C gm in samples representing strombolian and plinian eruption styles. Experimental studies have observed that larger clasts tend to have higher crystallinities as a result of slow air-cooling processes [18] . The low C gm of phreatomagmatic samples in this study support the general model that rapid quenching vastly reduces post-eruption microlite growth. Taking into account differences in clast size and microphenocryst content, groundmass crystallinities of phreatomagmatic materials (<35% C gm ) are distinguishable from magmatic volcanic products (>40% C gm ). However, fresh bulk samples appear to be more distinctive, with C wr of phreatomagmatic materials (<40%) significantly lower than other magmatic (>50%) volcanic deposits. The presence of phenocrysts causes a shift to higher crystallinity but appears to preserve the overall differences in eruption style in fresh to moderately altered samples ( Fig. 1b ). Therefore, crystallinity appears to be a robust proxy of cooling rate, with ‘magmatic’ explosive clasts showing evidence of greater microlite nucleation, owing to these materials remaining hotter for longer periods following fragmentation as compared with phreatomagmatic material. The relationship between cooling rate and crystallinity is well illustrated by a basaltic ignimbrite [23] from the Cascade volcanic arc ( Table 1 ). Crystallinity increases from 74 to 95% in weakly to moderately to densely welded ignimbrite. While basaltic ignimbrites are relatively rare in the geologic record on Earth, in silicic deposits the degree of welding is primarily controlled by bulk composition, emplacement temperature and accumulation rate. Densely welded ignimbrite deposits sinter following deposition and cool as a single unit rather than as discrete clasts. Such welding thus results in slower cooling rates and allows for a higher degree of groundmass crystallization [22] . Weathering and alteration effects on crystallinity The results of this study show that it is possible to understand and quantify the effect of weathering and alteration on crystallinity. Obtaining accurate crystallinity measurements for basaltic volcanic material becomes more challenging when significant quantities of alteration products are present, which is a scenario that is not unexpected on the Martian surface. Spectral data of bright regions on Mars suggest a prevalence of poorly crystalline or amorphous material, such as palagonite or nanophase iron oxides (npOx; [24] ). Poorly crystalline materials can have diffraction patterns that are not easily differentiated from those of true amorphous materials (for example, basaltic glass; Fig. 3 ). While basaltic glass creates one amorphous hump between ~15 and 35° 2 θ , palagonite, hisingerite, ferrihydrite and poorly crystalline aluminosilicates produce a low-angle rise at 4–10° 2 θ , with a weaker amorphous hump at (variable) higher angles ( Fig. 3 ) [25] , [26] . In low proportions, the broad low-angle peak characteristic of such materials may not be discernible. Weathering processes and low-temperature hydrothermal alteration may affect the interpretation of XRD patterns since devitrification of the glass component will increase crystallinity, and alteration of crystalline components to clays and other partially amorphous components will yield lower crystallinity measurements. In addition, the precipitation of calcite and zeolites will result in an increased crystallinity. 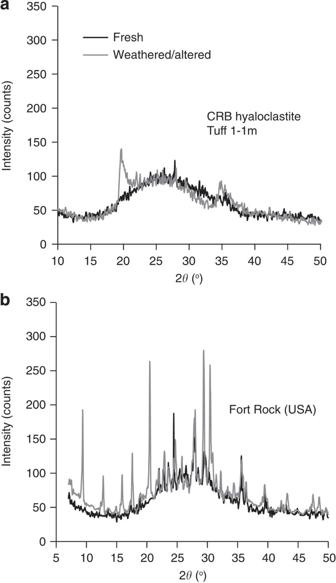Figure 3: Effects of alteration. Comparison between relatively fresh and weathered/altered samples from the same localities for phreatomagmatic samples. (a) Phreatomagmatic Columbia River basalt hyaloclastite fresh-picked glass (black line) and palagonitized bulk analysis (grey line). (b) Whole-rock analyses of weathered (grey line) and fresh (black line) tuffaceous material from Fort Rock (USA). An increase in peak intensity relative to that of the amorphous hump between 10–40° 2θin weathered/altered samples corresponds to increased crystallinity in both samples. Figure 3: Effects of alteration. Comparison between relatively fresh and weathered/altered samples from the same localities for phreatomagmatic samples. ( a ) Phreatomagmatic Columbia River basalt hyaloclastite fresh-picked glass (black line) and palagonitized bulk analysis (grey line). ( b ) Whole-rock analyses of weathered (grey line) and fresh (black line) tuffaceous material from Fort Rock (USA). An increase in peak intensity relative to that of the amorphous hump between 10–40° 2 θ in weathered/altered samples corresponds to increased crystallinity in both samples. Full size image Our results demonstrate that significant fractions of poorly crystalline alteration products in severely weathered/altered volcanic deposits can mask the original whole-rock crystallinity; however, the original C gm may still be preserved within groundmass glass fragments despite seemingly pervasive alteration. In light to moderately altered deposits, the whole-rock and groundmass crystallinities still reflect the broad distinctions between phreatomagmatic (<35%) and other magmatic (>35%) deposits ( Fig. 1b ). For example, in hyaloclastite tuffs within the Columbia River flood basalts, unaltered material from sample Tuff 1-1m is only ~8% crystalline, whereas a bulk analysis of the moderately palagonitized sample is ~30% crystalline, which are both clearly identifiable within the phreatomagmatic crystallinity range ( Figs 1 and 3 ). Similar variations may be observed in tuff deposits from Fort Rock, OR, where C wr increases from 22 to 47% with weathering; however, groundmass glass preserves nearly identical (~9–11%) crystallinities. More severe palagonitization of samples will blur the boundaries between these fields ( Fig. 1 and Table 1 ). However, in such cases, the alteration products will be at high enough proportions for their presence to be identifiable in the diffraction patterns ( Fig. 3 ) necessitating screening of results before interpretation. Bulk analyses of the severely weathered 122 BC plinian deposits from Mt. Etna generally yield higher crystallinities (by only 5–15%) than analyses of their fresher equivalents, whereas groundmass separates suggest a decrease from 46 to 36% as a result of greater weathering. These results suggest that in terms of measured crystallinities, alteration and weathering have varying and significant effects depending on the original crystal/glass content and style of alteration within volcanic products, but that C gm , even in severely altered samples, and random bulk crystallinity in light to moderately altered samples still preserves the broadly defined eruption styles. To successfully transfer this technique from Earth to Mars, several important considerations must be addressed, including sampling strategies, environmental factors and alteration processes. As previously demonstrated ( Fig. 1b ), random bulk and groundmass crystallinities in fresh to moderately altered eruptive products record the same distinction between phreatomagmatic and ‘magmatic’ eruption styles. This observation is critical to the applicability of this technique as a remote tool because it is not possible to separate groundmass from crystals using current remote sampling techniques [21] , and as a result, the Curiosity rover analyses are of bulk samples at the sub-125-μm sieve fraction. Hence, although the variations between eruption styles are defined by groundmass crystallization, this translates to the results of the random bulk (whole rock) analysis, and is therefore comparable to the MSL Curiosity rover sampling methodology [21] . Note that this does not discount the possibility that extremely high phenocryst contents in a phreatomagmatic deposit could skew results into the ‘magmatic’ crystallinity range. However, such deposits are rare on Earth ( Fig. 1b ). While the same styles of basaltic explosive eruptions are interpreted to exist on Mars (for example, phreatomagmatic, strombolian and plinian), differences in the Martian environment will impact eruption dynamics and ultimately crystallization of erupted materials [1] . Of particular significance to this study is the effect of lower atmospheric pressure on Mars (600 Pa average surface pressure) compared with Earth (101.3 kPa at sea level). A lower atmospheric pressure results in a 300 times decrease in the density of the erupted gas, decreasing the size of transportable particles on Mars by a factor of ~100 compared with Earth [1] . However, the lower atmospheric pressure also results in a 1.5 times increase in gas velocity and an increase in magma fragmentation such that explosive eruptions result in a greater dispersal of finer pyroclastic material on Mars compared with Earth with particles transported in eruption clouds predominantly sub-centimetre in diameter [1] . The overall decrease in clast size in Martian explosive volcanism particularly affects groundmass crystallization in air-cooled pyroclasts since cooling times are proportional, and cooling rates are inversely proportional, to the particle radius [27] . Assuming a spherical cooling model, particles <~1 cm rapidly re-equilibrate with their surroundings and remain in thermal equilibrium with the erupted gas in which they are entrained [1] , [27] . The cooling rate of small (<1 cm) erupted particles therefore is controlled by the cooling rate of the eruption plume they are in equilibrium with. Numerical simulations of a near-vent gas thrust model transitioning to a convective plume [27] , [28] modified for Martian atmospheric pressure and temperature [29] , eruption velocities and vent diameters [1] , and magma composition [30] ( Supplementary Table 1 ) are coupled with cooling rate–crystallization rate relationships above an estimated glass transition temperature of ~730 °C (refs. 18 , 31 ) to reconstruct syn-eruptive groundmass crystallization during plinian eruptions on Mars (see Supplementary Discussion 1 for details of numerical modelling). Modelled total syn-eruptive groundmass crystallization varies from 20 to 30% depending on particle sizes (1–5 mm radius), vent geometry and eruption velocities, for cooling times from ~25 to 200 s. Numerical simulations indicate that despite the lower atmospheric pressure and smaller particle sizes, cooling is buffered within the eruption plume, still allowing for significant groundmass crystallization. As rapid cooling rates and times associated with phreatomagmatic eruptive processes are not greatly affected by the change to Martian conditions there remains a measureable, if reduced, difference in crystallization between eruption styles, with syn-eruptive groundmass crystallization during plinian style increasing C gm by 20–30% compared with similar magma erupting phreatomagmatically. Larger clasts (> ~1 cm radius) that are modelled to rapidly fall out of the eruption plume have syn-eruptive C gm of >30%, resulting from slow conductive cooling of the clast interiors. Over geologic timescales, glass is a metastable material subject to alteration processes such as hydration and devitrification [32] . Although alteration of amorphous glass may result in the formation of crystalline materials (for example, zeolites), a by-product of both hydrothermal alteration and chemical weathering of glass on Mars is the formation of npOx. NpOx is an amorphous Fe-bearing constituent that may include haematite, goethite, ferrihydrite, hisingerite, schwertmanite, akaganeite and the Fe 3+ -rich particles that pigment iddingsite and palagonite, and is presently not distinguished from glass based on remote XRD analysis [33] , [34] , [35] , [36] , [37] , [38] , [39] . Alteration of glass is considered to be one of the primary means of npOx formation in Martian volcanic deposits [33] , [34] , [35] , [36] , [37] . However, npOx may also form from the dissolution of jarosite, a hydrous, K- and Fe-bearing sulfate [40] . While severe alteration of glass in Earth-based analogues results in an increase in crystallinity ( Fig. 1 ), from the assumption that npOx is predominantly derived from glass, the presence of significant amorphous npOx as an alteration product of glass on Mars should mitigate the effect of alteration on crystallinity measurements and the interpretation of eruptive processes. Although there is an absence of XRD data for Martian volcanic rocks, miniature thermal emission spectrometer (Mini-TES) analysis of pyroclastic rocks at Home Plate in Gusev crater, Mars, indicate a significant component of a material similar to basaltic glass (20–45%; refs 30 , 34 ). In contrast, Mössbauer spectroscopy results indicate a high proportion (27–29%) of npOx (absent from the Mini-TES results), suggesting that npOx may appear spectrally similar to basaltic glass using Mini-TES [30] . However, from the assumption that amorphous npOx is primarily derived from basaltic glass, the proportion of npOx may provide a means of estimating primary glass content even in severely altered volcanic rocks. A C wr of 55–80% from Mini-TES analysis of pyroclastic rocks in Gusev crater is consistent with a strombolian or plinian ‘magmatic’ eruption style, based on our methodology, rather than water/ice-driven phreatomagmatism [30] , [34] . However, high proportions of secondary silicate phases (up to ~25%) identified in some of the Home Plate mini-TES results may imply severe alteration and an underestimation of the glass content. New XRD data from the MSL Curiosity rover [38] processed using the calibration routine of this study indicate that the sediment making up the Rocknest sand shadow has a crystallinity of 52–54% ( Fig. 4 ) (compared with independent estimates from XRD [38] and mass balance [33] approaches, yielding 73±14% and 55% crystallinity, respectively). A calculation of the amorphous component chemical composition from a combination of CheMin and alpha particle X-ray spectrometer analysis on the Rocknest sand shadow sediment indicates a low-SiO 2 (37.2 wt%) component [33] . This is consistent with deconvolution of XRD patterns that indicate a best-fit to the CheMin XRD data with a ‘Gusev-composition basaltic glass [38] .’ Although multiple lines of evidence suggest the presence of a basaltic glass component, the origin and nature of this amorphous component is unknown [39] . Both volcanic eruptions and impacts have the potential to widely distribute glass on the surface of Mars [41] , [42] . Recent experimental work suggests a correlation between glass composition and the shape of the diffuse amorphous peak as analysed by XRD [43] . Several different types of impact glass are predicted on the Martian surface including proximal, low-SiO 2 (45–60 wt%) and distal tektite-like, high-SiO 2 (60–75 wt%) glass [41] . While distally deposited high-SiO 2 glass should produce an XRD pattern distinct from basaltic volcanic glass, low-SiO 2 proximal impact glass may be indistinguishable from basaltic volcanic glass [43] . As both basaltic impact glass and volcanic glass have the potential for distribution on the Martian surface, for now both remain a potential source of the amorphous component in the Rocknest sand shadow. 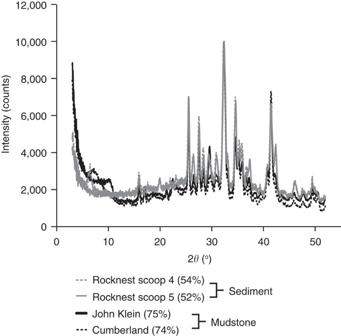Figure 4: Mars XRD patterns. XRD patterns of Rocknest sediment (scoops 4 and 5) and Yellowknife Bay mudstone rocks (John Klein and Cumberland) from Gusev crater, Mars, collected from the CheMin instrument on the Curiosity rover38,39. Bragg peaks in the diffraction pattern represent the crystalline component while the broad hump between ~10 and 40° 2θis characteristic of the amorphous component. Increasing crystallinity is reflected by relatively higher peak intensity compared with the broad hump of the amorphous component. Calculated bulk crystallinity from this study is indicated in parentheses. Figure 4: Mars XRD patterns. XRD patterns of Rocknest sediment (scoops 4 and 5) and Yellowknife Bay mudstone rocks (John Klein and Cumberland) from Gusev crater, Mars, collected from the CheMin instrument on the Curiosity rover [38] , [39] . Bragg peaks in the diffraction pattern represent the crystalline component while the broad hump between ~10 and 40° 2 θ is characteristic of the amorphous component. Increasing crystallinity is reflected by relatively higher peak intensity compared with the broad hump of the amorphous component. Calculated bulk crystallinity from this study is indicated in parentheses. Full size image The Rocknest sand shadow crystallinity estimate (52–54%) is significantly lower than the calculated crystallinity of Martian mudstones (John Klein and Cumberland) at Yellowknife Bay (Gale Crater) [39] (74–75%) using the same procedure, and is dominated by a basaltic mineral assemblage of plagioclase, olivine and pyroxene ( Fig. 4 ) [33] , indicating a potential source distinctive from that of the sediments comprising the mudstone rocks. With an understanding that the source of the amorphous component is debatable, based on the methodology developed here and the similarity in crystallinity and mineralogy between the Rocknest sand shadow sediment and the basaltic pyroclastic rocks of Gusev crater, we suggest that X-ray results are consistent with a relatively high proportion of basaltic glass indicating potentially widely distributed strombolian or plinian volcanic eruptive material on the surface of Mars [30] , [33] . This interpretation is consistent with the greater anticipated dispersal of explosive volcanic deposits on Mars [1] and prior observations regarding the widespread similarity between Martian soil and sediment [33] . In summary, application of our calibrated crystallinity technique provides a broadly applicable remote tool for quantifying the amorphous content of both sediments and rocks, and for potentially characterizing juvenile volcanic eruption styles and magma–water interaction on Earth and Mars. X-ray diffraction All analyses in this study were conducted using a Siemens D500 X-ray diffractometer at Washington State University with a CuKα source ( λ =1.54184 Å) operated at 35 kV and 30 mA. Samples (1–2 g) were powdered to a uniform particle size of ~20 μm, allowing for consistent and smooth sample preparation on glass plates (~0.1 g of material was used for sample mounts to ensure no interference from the substrate glass plate). Analyses were primarily conducted from 10 to 50° 2 θ at 0.03° steps and with 3.0 s dwell times (on select samples, data were collected down to 2° 2 θ to examine for low-angle peaks associated with alteration products; Fig. 3 ). Two incident beam slits and one diffracted beam slit were each positioned at 1°, followed by a diffracted beam graphite crystal monochronometer (0.05°). Using MDI JADE 8 software, diffractograms were processed with a 35-pt Savitzky–Golay smoothing filter to reduce background. Integrated counts were calculated above both cubic spline and linear backgrounds. The area above the linear background includes both the amorphous curve and crystalline peaks, whereas the integrated area above the cubic spline curve, applied to the base of the crystalline peaks, effectively eliminates the amorphous component and represents only the amount of crystalline material ( Fig. 2 ). Thus, the ratio of this ‘crystalline’ area over ‘total’ area, multiplied by 100%, provides a relative percent crystallinity ( RC (%)) of a sample (equation 1; ref. 22 ). where A CS and A L represent the integrated counts above the cubic spline and linear backgrounds, respectively. Crystallinity calibration In order to determine crystallinity values from RC(%), a calibration curve was constructed using samples of known crystallinity. Powder mixtures were created with varying weight percents of 100% crystalline material and 100% amorphous material (a glass plate) in order to mimic basalts of varying crystallinities ( Fig. 5 ). Two mixture series were created with one using a ‘natural’ gabbro and the other using a ‘synthetic’ gabbro, the latter created by powdering and mixing by weight single coarse samples of plagioclase (50%), orthopyroxene (40%) and olivine (10%). The two calibration curves deviate only slightly at high crystallinities, suggesting that the natural gabbro is probably not completely crystalline. Both curves record artificially high relative crystallinities (~10%) at low true crystallinity, which is a result of increased background interference associated with low count rates for amorphous materials ( Fig. 5 ). The ‘synthetic’ gabbro calibration was used in all subsequent calculations. 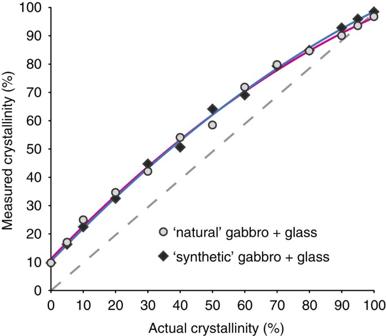Figure 5: Crystallinity calibration curves. Measured crystallinities, determined by XRD analysis, plotted against the samples’ known crystallinities. Known crystallinities are determined from mixing proportions of gabbro and glass. Both the ‘synthetic’ gabbro powder series and the ‘natural’ gabbro powder series yield best-fit curves, blue and purple lines respectively, that nearly align, and are both close to the 1:1 line (dashed grey line). The calibration curve is defined in terms of crystallinity as follows: Figure 5: Crystallinity calibration curves. Measured crystallinities, determined by XRD analysis, plotted against the samples’ known crystallinities. Known crystallinities are determined from mixing proportions of gabbro and glass. Both the ‘synthetic’ gabbro powder series and the ‘natural’ gabbro powder series yield best-fit curves, blue and purple lines respectively, that nearly align, and are both close to the 1:1 line (dashed grey line). Full size image where C (%) and RC (%) are the calibrated crystallinity and relative crystallinity, respectively. The calibrated methodology applied here for determining crystallinity is not a new approach. However, the application of this methodology as a new remote tool for determining volcanic eruption style is novel. Analysis of natural samples Whole-rock and groundmass crystallinities were determined from 17 eruptions of various styles. While the results discussed here focus on C gm for remote applications, it is important to relate whole rock and C gms since the physical separation of these different crystallinity measurements is not feasible during remote studies. Locations and descriptions of all samples are listed in Table 1 . Multiple analyses were conducted from each sample to investigate groundmass versus whole-rock crystallinity as well as the effects of weathering. In addition, a limited number of repeat analyses were conducted to test reproducibility and homogeneity of samples, indicated by trial number (1, 2 and 3) in Table 1 . A number of lava flows were also analysed to (1) provide a relative check of cooling rates and (2) to confirm that the amorphous substrate the samples are mounted on does not influence analyses. Massive Columbia River flood basalt lavas are nearly completely crystalline, with crystallinities varying from 80 to 98%, thus verifying that the sample mount substrate does not compromise the crystallinity calculations. In comparison with the slowly cooled Columbia River flood basalts, relatively glassy samples of smaller lava flows from Mt. Etna have substantially reduced crystallinities of 60–72%. XRD data from Mars sediment samples taken at the Rocknest sand shadow in Gale Crater (scoops 4 and 5; refs 33 , 38 ) and mudstones from Yellowknife Bay [39] were processed using our calibrated technique to determine the proportion of amorphous material. In contrast to the Siemens D500 that operates in reflection geometry mode with a CuKα X-ray source, the CheMin instrument operates in transmission geometry with a CoKα X-ray source [38] . While the absolute positions of peaks will vary as a result of the differences between wavelengths of CuKα and CoKα X-rays, overall differences in intensity will be relatively minor. As a result, crystallinities estimated from our calibrated approach, despite the differences in instruments, are expected to produce comparable results irrespective of the XRD instrument. How to cite this article : Wall, K. T. et al . Determining volcanic eruption styles on Earth and Mars from crystallinity measurements. Nat. Commun. 5:5090 doi: 10.1038/ncomms6090 (2014).